The role of maternal-specific H3K9me3 modification in establishing imprinted X-chromosome inactivation and embryogenesis in mice Maintaining a single active X-chromosome by repressing Xist is crucial for embryonic development in mice. Although the Xist activator RNF12/RLIM is present as a maternal factor, maternal Xist (Xm- Xist ) is repressed during preimplantation phases to establish imprinted X-chromosome inactivation (XCI). Here we show, using a highly reproducible chromatin immunoprecipitation method that facilitates chromatin analysis of preimplantation embryos, that H3K9me3 is enriched at the Xist promoter region, preventing Xm- Xist activation by RNF12. The high levels of H3K9me3 at the Xist promoter region are lost in embryonic stem (ES) cells, and ES-cloned embryos show RNF12-dependent Xist expression. Moreover, lack of Xm-XCI in the trophectoderm, rather than loss of paternally expressed imprinted genes, is the primary cause of embryonic lethality in 70–80% of parthenogenotes immediately after implantation. This study reveals that H3K9me3 is involved in the imprinting that silences Xm- Xist . Our findings highlight the role of maternal-specific H3K9me3 modification in embryo development. To maintain proper dosage compensation in mammals, one of the two X chromosomes in the female is inactivated [1] , [2] . In establishment of X-chromosome inactivation (XCI), a large non-coding RNA, Xist , is expressed and this non-coding RNA then covers the entire X chromosome in cis [1] , [2] , [3] . In mice, two types of XCI occur during female embryonic development. One type involves random XCI, which is observed in cells derived from epiblasts, and one of the two X chromosomes (paternal or maternal) is randomly inactivated. The other involves imprinted XCI (iXCI), which is observed in extra-embryonic tissues and causes XCI of the paternal X chromosome (Xp) [4] . The initiation of iXCI begins at early preimplantation in embryos and Xp- Xist is expressed around the four-cell stage [1] . A recent study showed that a maternal factor, the E3 ubiquitin ligase RNF12, is the primary factor responsible for Xp- Xist activation [5] . Interestingly, although RNF12 is abundant as a maternal factor in oocytes, Xm- Xist is not expressed. Moreover, maternal Xist (Xm- Xist )-specific imprints, which are refractory to the Xm- Xist activation induced by RNF12, are imposed during oogenesis [6] . Xist expression analysis using de novo DNA methyltransferase ( Dnmt3a / b ) maternal knockout mice demonstrated that Xist expression during preimplantation is independent of DNA methylation [7] , implying that other epigenetic factors are associated with Xm- Xist silencing. However, the nature of these Xm-specific epigenetic modifications is unknown. A gene-knockout study demonstrated that loss of Xp -Xist expression critically affects postimplantation female development due to lack of iXCI, which causes overexpression of X-linked genes in extra-embryonic tissues [8] . Similar to the phenotype observed in Xp- Xist -knockout mice, parthenogenetic embryos (PEs) composed of two X chromosomes show increased expression of X-linked genes, as compared with fertilized females, because of the low expression of Xist [9] . One of the interesting phenomena observed in PEs is the dramatic developmental failure that occurs immediately after implantation. Around 70–80% of embryos die before embryonic day (E) 9.5, which is the limit of development for PEs [10] . However, it is unknown whether the primary cause of rapid developmental failure in postimplantation PEs is the loss of iXCI or the loss of expression of autosomal paternally imprinted genes [11] , [12] . The global epigenetic asymmetry of parental genomes in zygotes is retained during early preimplantation phases in mice and changes in gene expression occur in discrete stages to confer totipotency [13] , [14] . Interestingly, transcriptionally repressive marks, such as histone H3 lysine 9 di-/trimethylation (H3K9me2/3), are specifically imposed on maternal genomes at the zygote stage [13] . Although the regulation of imprinted genes mostly depends on DNA methylation, some imprinted genes are regulated by these histone modifications [15] , [16] . Thus, Xm- Xist silencing machinery may be associated with histone modifications. Here we reveal that silencing of Xm- Xist in preimplantation embryos involves modification of H3K9me3. By using a new chromatin immunoprecipitation (ChIP) method that facilitates chromatin analysis in preimplantation embryos, we show that the Xist promoter on the Xm is highly enriched for H3K9me3 at the four-cell stage. This enrichment is lost in the morula and in male embryonic stem (ES) cells. Furthermore, we demonstrate that early loss of H3K9me3 at the Xist promoter leads to precocious Xm- Xist activation in a Rnf12-dependent manner. Moreover, we demonstrate that establishment of Xm-XCI in the trophectoderm allows PEs to develop at the postimplantation stage without the expression of paternally imprinted genes on autosomes. Therefore, these data indicate that the primary cause of embryonic lethality immediately after implantation in most PEs is loss of XCI rather than loss of the expression of paternally imprinted genes located on autosomes. Our study revealed that silencing of Xm- Xist by imprinting to establish iXCI involves H3K9me3, and this finding is expected to resolve the longstanding issues that have limited our general understanding of XCI in mice. Changes in histone modifications cause Xm- Xist derepression Histone repressive marks, such as H3K9me2/3 and H3K27me3, are specifically imposed on maternal genomes [13] . To investigate the role of maternal-specific modifications in imprinted Xist expression, we focused on Kdm3a and Kdm4b , which encode histone demethylases specific for H3K9me1/2 and H3K9me3 (refs 17 , 18 ), respectively. Reverse transcription–PCR analysis showed that oocytes express low levels of Kdm3a and Kdm4b ( Supplementary Fig. 1 ). Immunofluorescence (IF) analyses revealed that zygotes injected with polyadenylated Kdm3a and Kdm4b messenger RNAs expressed significantly lower levels of maternal H3K9me2 and H3K9me3, respectively ( Fig. 1a–d ). Ectopic expression of Kdm3a and Kdm4b did not affect H3K9me3 or H3K9me2 marks, respectively ( Supplementary Fig. 2 ). We reasoned that if Xm-specific modifications that prevent Xist activation were erased by these epigenetic modifiers, Xm- Xist would be expressed at the four-cell stage, which is when Xp- Xist expression commences. 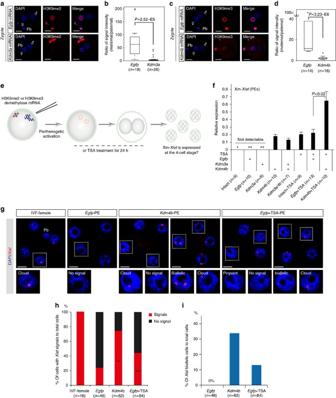Figure 1: Alterations in histone modifications derepress Xm-Xistexpression. (a–d) Oocytes injected withKdm3a(a,b),Kdm4b(c,d) orEgfpmRNAs were subjected to ICSI. After 7–8 h, embryos were fixed and analysed for H3K9me2 (a) and H3K9me3 (c) using IF. Nuclei stained with 4′,6-diamidino-2-phenylindole (DAPI) are shown in blue. Representative images are presented on the left. The box-and-whisker plot shows the ratio of maternal to paternal signal intensities. The horizontal line indicates the median. TheP-values were calculated using the Mann–WhitneyU-test (U-test). Pb, polar body;n, number of embryos analysed (b,d). (e) Schema of the generation of PEs with altered histone modifications. To examine the effects of histone demethylation on Xm-Xistexpression, either H3K9me2 demethylase (Kdm3a) or H3K9me3 demethylase (Kdm4b) mRNAs were injected into MII oocytes that were then activated. To assess the effects of inhibition of histone deacetylation on Xm-Xistexpression, oocytes were activated and incubated in the presence of TSA for 24 h. After 48 h, ten four-cell PEs were pooled and analysed as one biological replicate using qPCR. (f) Analysis of Xm-Xistexpression at the four-cell stage. The expression level of Xm-Xistin female embryos derived from IVF was defined as 1. One or two asterisks indicate Xm-Xistexpression in one or two replicates, respectively. TheP-values were determined using Student’st-tests. Error bars indicate the mean±s.e.m. (g–i)XistFISH analysis ofKdm4b- andEgfp+TSA-PEs at the four-cell stage. (g) Representative images of FISH results. (h) Ratio of cells withXistsignal to the total number of cells.n, number of interphase cells analysed. (i) Ratio of cells with biallelic expression to total cells. The detailed FISH results are shown inSupplementary Table 1. Scale bars, 20 μm. Figure 1: Alterations in histone modifications derepress Xm- Xist expression. ( a – d ) Oocytes injected with Kdm3a ( a , b ), Kdm4b ( c , d ) or Egfp mRNAs were subjected to ICSI. After 7–8 h, embryos were fixed and analysed for H3K9me2 ( a ) and H3K9me3 ( c ) using IF. Nuclei stained with 4′,6-diamidino-2-phenylindole (DAPI) are shown in blue. Representative images are presented on the left. The box-and-whisker plot shows the ratio of maternal to paternal signal intensities. The horizontal line indicates the median. The P -values were calculated using the Mann–Whitney U -test ( U -test). Pb, polar body; n , number of embryos analysed ( b , d ). ( e ) Schema of the generation of PEs with altered histone modifications. To examine the effects of histone demethylation on Xm- Xist expression, either H3K9me2 demethylase ( Kdm3a ) or H3K9me3 demethylase ( Kdm4b ) mRNAs were injected into MII oocytes that were then activated. To assess the effects of inhibition of histone deacetylation on Xm- Xist expression, oocytes were activated and incubated in the presence of TSA for 24 h. After 48 h, ten four-cell PEs were pooled and analysed as one biological replicate using qPCR. ( f ) Analysis of Xm- Xist expression at the four-cell stage. The expression level of Xm- Xist in female embryos derived from IVF was defined as 1. One or two asterisks indicate Xm- Xist expression in one or two replicates, respectively. The P -values were determined using Student’s t -tests. Error bars indicate the mean±s.e.m. ( g – i ) Xist FISH analysis of Kdm4b - and Egfp +TSA-PEs at the four-cell stage. ( g ) Representative images of FISH results. ( h ) Ratio of cells with Xist signal to the total number of cells. n , number of interphase cells analysed. ( i ) Ratio of cells with biallelic expression to total cells. The detailed FISH results are shown in Supplementary Table 1 . Scale bars, 20 μm. Full size image To facilitate analysis of Xm- Xist expression, we used PEs ( Fig. 1e ). PEs possess two copies of Xm, and Xm- Xist is never expressed at the four-cell stage [19] . Xm- Xist expression in four-cell PEs, cultured for 48 h, was determined using quantitative real-time PCR (qPCR). Consistent with a previous report [19] , Xm- Xist was not detectably expressed in most intact (not injected) PEs and PEs injected with Egfp mRNA ( Egfp -PEs; Fig. 1f ). Approximately 75% of PEs injected with Kdm3a mRNA ( Kdm3a -PEs) did not detectably express Xist . However, Xm- Xist expression was detected in all PEs injected with Kdm4b mRNA ( Kdm4b -PEs; Fig. 1f ), suggesting that H3K9me3 demethylation caused Xm- Xist derepression. We next assessed the effects of a histone deacetylase inhibitor, trichostatin A (TSA), on Xm- Xist expression. TSA-treated PEs (Intact+TSA-PEs and Egfp +TSA-PEs) also activated Xm- Xist ( Fig. 1f ). No significant changes were detected in Xm- Xist expression levels between Kdm4b -PEs and Egfp +TSA-PEs. However, although co-injection with Kdm4b and Kdm3a mRNAs did not increase Xm- Xist expression levels as compared with Kdm4b -PEs, a combination of TSA and Kdm4b -mRNA significantly increased Xm- Xist expression as compared with Egfp +TSA-PEs (2.9-fold, P <0.04, Student’s t -test; Fig. 1f ). Moreover, derepression of Xm- Xist transcription occurred in the absence of Rnf12 overexpression ( Supplementary Fig. 3 ), and Jpx and Ftx , which have been identified as Xist activators [2] , were not expressed at the four-cell stage. These results showed that KDM4B- and TSA-mediated Xm- Xist derepression was not involved in the abnormal expression of known Xist activators. Next, we examined Xm- Xist derepression states at the single-cell level by fluorescence in situ hybridisation (FISH) of Xist RNA. Consistent with the qPCR results, Xm- Xist signals were significantly increased in Egfp +TSA- and Kdm4b -PEs ( Fig. 1g,h and Supplementary Table 1 ). However, neither TSA treatment nor Kdm4b overexpression consistently activated Xm- Xist in all cells ( Fig. 1g,h ). FISH analysis also revealed Xist biallelic cells in Kdm4b - and Egfp +TSA-PEs ( Kdm4b -PEs: 34% and Egfp +TSA-PEs: 13%; Fig. 1g,i ). Taken together, these results indicated that Kdm4b overexpression and TSA treatment induced Xm- Xist derepression at the same developmental stage as Xp- Xist activation. Xm- Xist transcripts establish XCI at the blastocyst stage To investigate whether Xm- Xist transcripts from the four-cell stage induced XCI in late preimplantation stages, we cultured Kdm4b -, Egfp +TSA- and Kdm4b +TSA-PEs until the blastocyst stage. 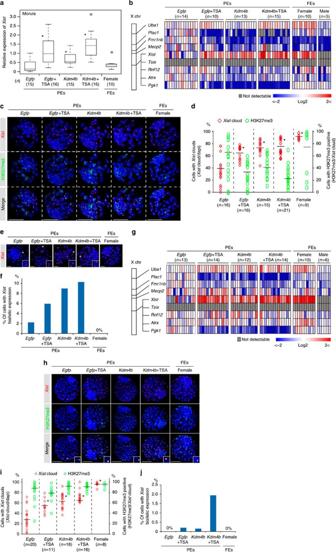Figure 2: Global XCI andXistexpression states of Xm at late preimplantation stages. (a) Analysis ofXistexpression using qPCR of individual embryos in the morula. An asterisk indicatesP<0.05 (Student’st-test) compared withEgfp-PEs. FEs, fertilized embryos. (b) Large-scale qPCR analysis ofXistand eight X-linked genes in individual blastocysts after culturing for 96 h. Coloured bars indicate expression levels. (c,d) IF (H3K27me3, green) combined with RNA FISH (Xist, red) analysis in 96-h blastocyst stage. 4′,6-diamidino-2-phenylindole (DAPI)-stained nuclei are shown in blue. (c) Representative confocal projection. Scale bars, 50 μm. (d) The graph showsXistexpression and H3K27me3 modification states in individual embryos. The horizontal axis indicates the average percentage in the group. *P<3.1 × 10−28(Fisher’s exact test).n, number of embryos analysed. (e,f) Xm-Xistbiallelic expression states in PEs at 96 h. The asterisk indicates cells with biallelic expression. Scale bars, 20 μm. (f) Summary of the ratio of biallelic cells toXist-positive cells in 96-h blastocyst stage in each group. The number of cells is shown inSupplementary Table 3. (g) qPCR analysis ofXistand eight X-linked genes in individual blastocysts after culturing for 120 h. (h,i) IF (H3K27me3, green) combined with RNA FISH (Xist, red) analysis in 120 h blastocysts. *P<5.4 × 10−23(Fisher’s exact test). Scale bars, 50 μm. (j) The ratio of biallelic cells toXist-positive cells in 120 h blastocysts. In qPCR analysis, the average expression level of Xm-XistinEgfp-PEs was set as 1 (also see the Methods section).Gapdhandβ-actinwere used as internal controls. Data are summarized inSupplementary Table 4. Development into blastocysts occurred in >80% of PEs in all groups ( Supplementary Table 2 ). At the morula stage (72 h), although Egfp -PEs initiated Xm- Xist expression, the levels of Xist expression were significantly lower compared with those in Kdm4b -injected and/or TSA-treated PEs ( Fig. 2a ). At the 96-h blastocyst stage, we examined the expression levels of Xist and X-linked genes ( Tsix , Rnf12 , Pgk1 , Fmr1nb , Atrx , Uba1 , Mecp2 and Plac1 ) in individual embryos. The significant upregulation of Xist observed in PEs that had been injected with Kdm4b mRNA and/or TSA continued in 96-h blastocyst stage ( Fig. 2b ). In PEs exhibiting Xm- Xist upregulation, Tsix expression was not detectable and Rnf12 was not overexpressed as compared with Egfp -PEs ( Fig. 2b ). The average expression levels of Pgk1 , Plac1 and Fmr1nb in Kdm4b -overexpressing or TSA-treated PE groups were significantly reduced ( Supplementary Fig. 4a ). However, single embryos in the same group exhibited heterogeneity in the expression levels of these targets ( Fig. 2b ). Moreover, although Xm- Xist was not overexpressed in Kdm4b -overexpressing or TSA-treated PE groups compared with levels seen in female fertilized embryos (FEs), the levels of Plac1 and Pgk1 were strongly downregulated in Kdm4b -, Egfp +TSA- and Kdm4b +TSA groups ( Fig. 2b ). These results suggested that Xm- Xist expression states differed at the single-cell level in individual embryos. Figure 2: Global XCI and Xist expression states of Xm at late preimplantation stages. ( a ) Analysis of Xist expression using qPCR of individual embryos in the morula. An asterisk indicates P <0.05 (Student’s t -test) compared with Egfp -PEs. FEs, fertilized embryos. ( b ) Large-scale qPCR analysis of Xist and eight X-linked genes in individual blastocysts after culturing for 96 h. Coloured bars indicate expression levels. ( c , d ) IF (H3K27me3, green) combined with RNA FISH ( Xist , red) analysis in 96-h blastocyst stage. 4′,6-diamidino-2-phenylindole (DAPI)-stained nuclei are shown in blue. ( c ) Representative confocal projection. Scale bars, 50 μm. ( d ) The graph shows Xist expression and H3K27me3 modification states in individual embryos. The horizontal axis indicates the average percentage in the group. * P <3.1 × 10 −28 (Fisher’s exact test). n , number of embryos analysed. ( e , f ) Xm- Xist biallelic expression states in PEs at 96 h. The asterisk indicates cells with biallelic expression. Scale bars, 20 μm. ( f ) Summary of the ratio of biallelic cells to Xist -positive cells in 96-h blastocyst stage in each group. 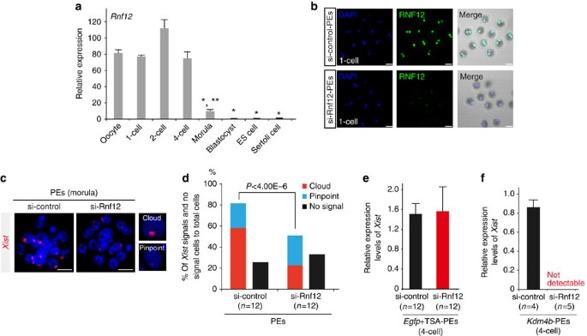Figure 3: RNF12 is required forXistexpression in various types of preimplantation embryos. (a)Rnf12expression profiles in preimplantation stages, ES cells and somatic cells. Ten oocytes (n=3), ten IVF-1 cells (n=3), ten IVF-2 cells (n=3) and five IVF-4 cells (n=3) were pooled. The expression level ofRnf12in the morula stage, as determined using qPCR, represents the average of 16 individual embryos. The numbers of ES and Sertoli cells represent the averages of three independent cell lines and male pups, respectively. The error bars indicate the mean±s.e.m. *P<0.004 compared with oocytes; **P<0.0001 compared with ES cells (Student’st-test). (b) IF analysis of RNF12 at the one-cell stage (green). Samples were fixed 11 h after parthenogenetic activation (18–19 h after siRNA injection). The same laser beam intensities were used to excite theRnf12-knockdown and control samples. 4′,6-diamidino-2-phenylindole (DAPI)-stained nuclei are shown in blue. Two independent experiments were conducted. Scale bars, 50 μm. (c,d)XistFISH analysis of si-Rnf12 PEs at the morula stage. At 72 h after activation, PEs injected with siRNA were analysed. Representative images of siRNA-treated embryos (c). Scale bars, 20 μm. The percentage of totalXist-positive signals and -negative cells to total cells in si-Rnf12 and si-control PEs. Biallelic expression was counted as two signals.n, number of embryos analysed (d). (e,f) qPCR analysis of Xm-Xistexpression at the four-cell stage of embryos treated with TSA (e) or injected withKdm4bmRNA (f). PEs derived from maternal si-Rnf12-treated oocytes. A detailed experimental scheme is shown inSupplementary Fig. 6d. A pool of eight to ten four-cell embryos represents one biological replicate. The number of cells is shown in Supplementary Table 3 . ( g ) qPCR analysis of Xist and eight X-linked genes in individual blastocysts after culturing for 120 h. ( h , i ) IF (H3K27me3, green) combined with RNA FISH ( Xist , red) analysis in 120 h blastocysts. * P <5.4 × 10 −23 (Fisher’s exact test). Scale bars, 50 μm. ( j ) The ratio of biallelic cells to Xist -positive cells in 120 h blastocysts. In qPCR analysis, the average expression level of Xm- Xist in Egfp -PEs was set as 1 (also see the Methods section). Gapdh and β-actin were used as internal controls. 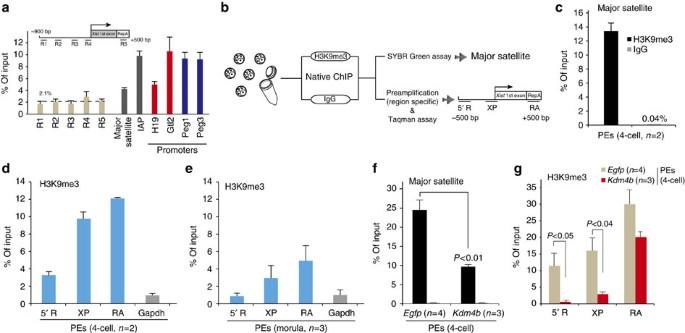Figure 4: H3K9me3 states at the Xm-Xistpromoter region in preimplantation embryos. (a) ChIP-qPCR analysis of Xp (sperm) atXist5′-regions, theH19,Gtl2,Peg1andPeg3promoter region, and regions in repetitive elements.n=2–4. Rabbit IgG was used as a negative control. The percentage of input for negative control DNA was >1% for all genes tested. The data were not normalized for local nucleosome occupancies. (b) Schematic representation of eChIP-qPCR analysis. H3K9me3 states at major satellite regions (c) and atXistregions and theGapdhpromoter region (d) in PEs at the four-cell stage. Two independent experiments were performed. In each experiment, 250 embryos were used. (e) H3K9me3 states at theXistandGapdhpromoter regions in morula-stage embryos. Three independent experiments were conducted and 40 embryos were used for each assay. H3K9me3 states in major satellite (f) andXistregions (g) inEgfp- andKdm4b-PEs at the four-cell stage. Three (Kdm4b-PEs) and four (Egfp-PEs) independent experiments were conducted. In each experiment, 170–250 embryos were prepared. The percentages of input for negative controls (IgG) were <0.2% (f) and 1.9% (g), respectively. Error bars indicate the mean±s.e.m. TheP-values were determined using Student’st-tests. Data are summarized in Supplementary Table 4 . Full size image To gain further insights into Xist expression states and repression of X-linked genes on Xm alleles, we conducted IF to detect the H3K27me3 state, which is a hallmark of XCI [20] , and performed Xist FISH analysis. The Xist RNA FISH probe recognizes Xist and Tsix . Therefore, the cloud state of the FISH signal defined Xist expression. Consistent with the qPCR results, the number of cells with Xist signals increased significantly in all Kdm4b -overexpressing or TSA-treated PEs ( Fig. 2c and Supplementary Table 3 ). However, in all Kdm4b -overexpressing or TSA-treated PEs, <45% of Xist cloud-containing cells had an H3K27me3 signal ( Fig. 2c,d and Supplementary Table 3 ). We also found that Xist biallelic cells were present in all PE groups ( Egfp -PEs: 2.2%, Egfp +TSA-PEs: 5.9%, Kdm4b -PEs: 9.0% and Kdm4b +TSA-PEs: 10.3%; Fig. 2e,f ). These results suggested that there were various Xm- Xist expression states present at the single-cell level, affecting the heterogeneity of X-linked genes, and that strong suppression of some X-linked genes in Kdm4b -overexpressing or TSA-treated PEs could be attributed to biallelic expression of Xm- Xist . As Kdm4b overexpression and TSA treatment did not affect the extent of H3K27me3 modification ( Supplementary Fig. 5 ), its acquisition in PEs may have been slightly delayed compared with that in FEs. In support of this notion, the developmental timing of PEs lags behind that of FEs [9] . Therefore, we extended the culture period to 120 h and again performed qPCR, IF and FISH analyses. As seen in 96-h blastocyst stage, qPCR analysis revealed that Plac1 and Pgk1 were significantly repressed in Kdm4b -overexpressing or TSA-treated PEs, although heterogeneity was observed ( Fig. 2g and Supplementary Fig. 4b ). However, Fmr1nb , which was significantly repressed in 96-h blastocyst stage of both Kdm4b - and TSA-treated groups, did not show marked suppression ( Fig. 2g and Supplementary Fig. 4b ), suggesting that Xist expression states were altered in 120 h blastocysts. In FISH and IF analysis, a significant increase in the number of Xist -positive cells was detected in Kdm4b -overexpressing and/or TSA-treated PEs, as compared with Egfp -PEs, after culture for 120 h ( Fig. 2h,i and Supplementary Table 4 ). There was a marked increase in the ratio of H3K27me3 spots to cloud Xist signals in blastocysts in all groups compared with that observed after 96 h of culture as follows: 88.1% in Egfp -PEs, 78.7% in Egfp +TSA-PEs, 91.8% in Kdm4b -PEs and 91.2% in Kdm4b +TSA-PEs ( Fig. 2h,i and Supplementary Table 4 ). Interestingly, >98% of the cells in the Xist cloud state exhibited monoallelic Xist expression in all groups at 120 h ( Fig. 2j ). Taken together, these results indicated that Kdm4b overexpression and TSA treatment induced global XCI of Xm in blastocysts and that the counting mechanism automatically functioned in late blastocysts, as has also been observed for Xp alleles [21] . KDM4B-mediated Xm -Xist expression depends on RNF12 During preimplantation phases, Xp- Xist expression is induced by maternal RNF12 (ref. 5 ). Thus, we investigated whether Xm- Xist expression also depended on RNF12. High Rnf12 expression levels were maintained until the four-cell stage (around 80-fold higher than in ES cells; Fig. 3a ). At the morula stage, although the expression level was significantly decreased compared with that in oocytes, Rnf12 expression was still more than ninefold higher than that in ES cells ( Fig. 3a ), indicating that maternal and early zygotic RNF12 may be critical for Xm- Xist activation. To examine the dependency of RNF12 on Xm- Xist expression, we inhibited maternal and zygotic RNF12 expression using Rnf12 -siRNA ( Supplementary Fig. 6a ). IF analysis at the one-cell stage showed a marked decline in RNF12 signal intensity in si- Rnf12 embryos compared with that in the si-control embryos ( Fig. 3b ). Significant repression by si- Rnf12 was maintained in the four-cell stage ( Supplementary Fig. 6b,c ). Using this knockdown system, we examined whether Xm- Xist activation was induced by RNF12 at the morula stage. Xist FISH analysis revealed that Xist signals (cloud and pinpoint) in PEs treated with si-Rnf12 were significantly reduced at the morula stage as compared with those observed in the controls (si-Rnf12: 50.0% versus si-control: 80.0%; Fig. 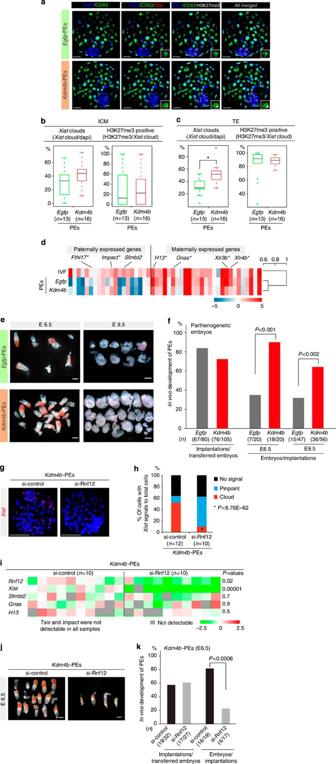Figure 5: Loss of Xm-XCI is the primary cause of developmental failure immediately after implantation in most PEs. (a) IF combined with FISH analysis of blastocysts inEgfp-PEs (upper panel) andKdm4b-PEs (lower panel). CDX2-positive cells were identified as belonging to the trophectoderm (TE). Representative pictures of Z-sections. 4′,6-diamidino-2-phenylindole (DAPI) (blue), CDX2 (green),Xist(red) and H3K27me3 (white). Scale bars, 20 μm. The rates of cells withXist(left) or H3K27me3 (right) in the inner cell mass (ICM) (b) and TE (c), respectively.n, number of embryos analysed. The number of cells analysed is shown inSupplementary Table 7. *P<4.3 × 10−23(Fisher’s exact test). (d) Expression states and clustering analysis of imprinted genes.Sfmbt2important for placentation and differentially expressed genes (asterisk) are shown. The scale bar indicates normalized values of log2. (e) Embryos with extra-embryonic tissues at E6.5 and E9.5 forKdm4b- andEgfp-PEs, respectively. Upper and lower images indicateEgfp- andKdm4b-PEs, respectively. Left and right column sides show E6.5 and E9.5, respectively. Scale bars, 200 μm (E6.5) and 500 μm (E9.5). (f) Summary of the developmental abilities ofKdm4b-PEs andEgfp-PEs at postimplantation stages (E6.5 and E9.5). Five and 12 independent recipients were analysed at E6.5 and E9.5, respectively. (g,h)Xistanalysis inRnf12-knockdown and controlKdm4b-PEs. Representative images of FISH analysis. Scale bars, 50 μm (g) andXistexpression states (h). (i) Expression of imprinted and X-linked genes inRnf12-knockdown and controlKdm4b-PEs.P-values were determined using Student’st-tests. (j) Embryos with extra-embryonic tissues at E6.5 inRnf12-knockdown and controlKdm4b-PEs. Scale bars, 200 μm. (k) Summary of the developmental ability ofRnf12-knockdown and controlKdm4b-PEs at E6.5. Five independent recipients were analysed. TheP-values were determined using Fisher’s exact test. 3c,d and Supplementary Table 5 ). Figure 3: RNF12 is required for Xist expression in various types of preimplantation embryos. ( a ) Rnf12 expression profiles in preimplantation stages, ES cells and somatic cells. Ten oocytes ( n =3), ten IVF-1 cells ( n =3), ten IVF-2 cells ( n =3) and five IVF-4 cells ( n =3) were pooled. The expression level of Rnf12 in the morula stage, as determined using qPCR, represents the average of 16 individual embryos. The numbers of ES and Sertoli cells represent the averages of three independent cell lines and male pups, respectively. The error bars indicate the mean±s.e.m. * P <0.004 compared with oocytes; ** P <0.0001 compared with ES cells (Student’s t -test). ( b ) IF analysis of RNF12 at the one-cell stage (green). Samples were fixed 11 h after parthenogenetic activation (18–19 h after siRNA injection). The same laser beam intensities were used to excite the Rnf12 -knockdown and control samples. 4′,6-diamidino-2-phenylindole (DAPI)-stained nuclei are shown in blue. Two independent experiments were conducted. Scale bars, 50 μm. ( c , d ) Xist FISH analysis of si-Rnf12 PEs at the morula stage. At 72 h after activation, PEs injected with siRNA were analysed. Representative images of siRNA-treated embryos ( c ). Scale bars, 20 μm. The percentage of total Xist -positive signals and -negative cells to total cells in si-Rnf12 and si-control PEs. Biallelic expression was counted as two signals. n , number of embryos analysed ( d ). ( e , f ) qPCR analysis of Xm- Xist expression at the four-cell stage of embryos treated with TSA ( e ) or injected with Kdm4b mRNA ( f ). PEs derived from maternal si-Rnf12-treated oocytes. A detailed experimental scheme is shown in Supplementary Fig. 6d . A pool of eight to ten four-cell embryos represents one biological replicate. Full size image Next, we examined whether Xm- Xist derepression from the four-cell stage by ectopic Kdm4b expression or TSA treatment was regulated by RNF12 ( Supplementary Fig. 6d ). Four-cell embryos of Kdm4b - or Egfp +TSA-PEs treated with si-Rnf12 were analysed by qPCR. Depletion of RNF12 did not affect Xm- Xist expression in Egfp +TSA-PEs compared with the si-control PEs ( Fig. 3e ), suggesting that factors other than RNF12 may contribute to histone acetylation-mediated Xm- Xist activation. This observation is consistent with results obtained using Rnf12 −/− mice, which demonstrated that Xist is activated by RNF12 and other unidentified factors [5] , [22] . In contrast, Xist expression in Kdm4b -PEs derived from oocytes treated with si- Rnf12 did not induce detectable expression of Xm- Xist ( Fig. 3f ). These results demonstrated that KDM4B-mediated Xm- Xist expression depended on RNF12 and suggested that H3K9me3 prevented the expression. Promoter demethylation of H3K9me3 causes Xm- Xist derepression As activation of Xist by RNF12 is essential for establishing iXCI [5] , we attempted to determine the mechanism responsible for the transcriptional derepression of Xm- Xist by KDM4B-mediated demethylation of H3K9me3. We first examined whether H3K9me3 levels were enriched at the Xp- Xist promoter region. Nucleosomes were extracted from the sperm genome ( Supplementary Fig. 7 ). ChIP-qPCR revealed the low H3K9me3 levels of Xp- Xist in the 5′-regions containing the major promoter for Xist expression (average: 2.1%; Fig. 4a ), as compared with those of the H19 , Gtl2 , Peg1 and Peg3 promoter loci (average: 8.5%) and regions in repetitive elements (intracisternal A-particles and major satellite DNAs; average: 7.0%), which are known to be associated with H3K9me3 (ref. 23 ). These results indicated that the Xist promoter region was hypomethylated in sperm, in agreement with Xp- Xist being expressed in early embryogenesis. Figure 4: H3K9me3 states at the Xm- Xist promoter region in preimplantation embryos. ( a ) ChIP-qPCR analysis of Xp (sperm) at Xist 5′-regions, the H19 , Gtl2 , Peg1 and Peg3 promoter region, and regions in repetitive elements. n =2–4. Rabbit IgG was used as a negative control. The percentage of input for negative control DNA was >1% for all genes tested. The data were not normalized for local nucleosome occupancies. ( b ) Schematic representation of eChIP-qPCR analysis. H3K9me3 states at major satellite regions ( c ) and at Xist regions and the Gapdh promoter region ( d ) in PEs at the four-cell stage. Two independent experiments were performed. In each experiment, 250 embryos were used. ( e ) H3K9me3 states at the Xist and Gapdh promoter regions in morula-stage embryos. Three independent experiments were conducted and 40 embryos were used for each assay. H3K9me3 states in major satellite ( f ) and Xist regions ( g ) in Egfp - and Kdm4b -PEs at the four-cell stage. Three ( Kdm4b -PEs) and four ( Egfp -PEs) independent experiments were conducted. In each experiment, 170–250 embryos were prepared. The percentages of input for negative controls (IgG) were <0.2% ( f ) and 1.9% ( g ), respectively. Error bars indicate the mean±s.e.m. The P -values were determined using Student’s t -tests. Full size image Preparing sufficient numbers of embryos or oocytes for ChIP combined with deep sequencing (ChIP-seq) analysis is problematic. Some ChIP-qPCR methods requiring small samples have been reported [24] ; however, most of these studies are based on a cross-linking ChIP method, in which the ChIP efficiency is lower than that of native ChIP methods [25] . Thus, we developed a new native ChIP method combined with a Taqman qPCR system for quantification of transcription in single cells (termed eChIP-qPCR) and focused on three loci at Xist 5′-regions containing the major promoter and repeat A, which is essential for establishment of iXCI [26] ( Fig. 4b ). We first tested whether the quantification system was biased by using diluted DNA from bulk ES cells. The results of ChIP-qPCR from pre-amplified DNA were comparable to those obtained without pre-amplification ( Supplementary Fig. 8 ). Using this system, we examined H3K9me3 states at three Xist regions and at Gapdh promoter regions (as a negative control) in PEs at the four-cell stage. We first investigated whether our eChIP method was efficient by examining major satellite repeats that have been identified as H3K9me3-rich regions in preimplantation embryos [23] . Consistent with a previous report, H3K9me3 was highly enriched at major satellite regions ( Fig. 4c ). The three Xist regions were also highly methylated compared with the Gapdh promoter region, as follows: 5′-R, 3.7-fold upregulated; XP, 9.8-fold upregulated; RA, 12.1-fold upregulated; ( Fig. 4d ). As Fig. 2a showed Xm- Xist spontaneous derepression at the morula stage, we next investigated whether H3K9me3 levels at the Xist promoter region were low at this stage. eChIP-aPCR analysis revealed that enrichment of H3K9me3 was markedly reduced compared with that at the Gapdh promoter region in the four-cell stage (5′-R, 0.83-fold upregulated; XP, 2.85-fold upregulated; RA, 4.8-fold upregulated; Fig. 4e ). These results suggested that demethylation at the promoter region was essential for Xm- Xist derepression. We then asked whether Xist promoter demethylation was involved in the Xm- Xist derepression observed in Kdm4b -PEs at the four-cell stage. The H3K9me3 levels at major satellite regions in Kdm4b -PEs were significantly reduced compared with those in Egfp -PEs ( Kdm4b -PEs: 9.74% versus Egfp -PEs: 24.63%, P <0.01, Student’s t -tests; Fig. 4f ). At three Xist regions, the H3K9me3 levels of the promoter region in Kdm4b -PEs were significantly reduced, as follows: 5′-R, Kdm4b -PEs: 0.84% versus Egfp -PEs: 11.48%, P <0.05, Student’s t -tests; XP, Kdm4b -PEs: 3.13% versus Egfp -PEs: 16.08%; P <0.04, Student’s t -tests; and RA, Kdm4b -PEs: 20.16% versus Egfp -PEs: 29.99%; Fig. 4g . Taken together, these results demonstrated that H3K9me3 at the promoter region protected Xm- Xist , preventing RNF12-mediated activation from the four-cell stage. We concluded that silencing of Xm- Xist by imprinting to establish iXCI involved H3K9me3. Maternal repressive H3K9me3 mark is absent in ES cells Previous studies have shown that Xist is ectopically expressed in embryos cloned from somatic and ES cells [27] , [28] . However, the cause of aberrant Xist expression in cloned embryos remains unknown. Given that high H3K9me3 levels at the promoter region in PEs are lost during development ( Fig. 4d,e ), we investigated whether the maternal repressive H3K9me3 mark was lost in ES cells and whether Xist in ES cells was permissive against RNF12 during oocyte-mediated reprogramming. To test this possibility, we first examined H3K9me3 states at Xist regions in various types of male ES cells, using published data [29] , [30] . The levels of H3K9me3 at Xist regions containing promoters in TT2 and E14 ES cell lines were low compared with those in positive control regions ( Supplementary Fig. 9 ). ChIP-seq analysis revealed that although ectopic expression of KDM4B in male ES cells induced global H3K9me3 demethylation ( Supplementary Fig. 10a–d ), it did not alter H3K9me3 levels at Xist regions. Moreover, these levels were low compared with those of a known H3K9me3-rich region ( Supplementary Fig. 10e ) [16] . Furthermore, the expression of Xist in cloned embryos was also not affected by ectopic expression of KDM4B ( Supplementary Fig. 10f ). These results indicated that the maternal repressive H3K9me3 mark was lost. To establish whether RNF12 is involved in Xist activation during oocyte-mediated reprogramming, oocytes treated with si- Rnf12 were used as recipients for nuclear transfer ( Supplementary Fig. 10g ). At the four-cell stage, derepression of Xist transcription in ES-cloned embryos depended on RNF12 (>50% repression in si- Rnf12 group; Supplementary Fig. 10h ). Taken together, these data indicated that the intrinsic H3K9me3 mark, which was essential for repression of Xist by RNF12, was lost during embryo development. This indicated that the primary cause of aberrant Xist expression in cloned embryos was involved in loss of intrinsic H3K9me3 at Xist regions. Effects of iXCI disruption on FEs The effects of Xm- Xist derepression on postimplantation development remain unclear. First, we asked whether ectopic Kdm4b expression caused Xm- Xist derepression in FEs. Kdm4b -FEs developed into blastocysts with high efficiency (>80% of two-cell embryos; Supplementary Table 6 ). At the 96-h blastocyst stage, Xist transcription was derepressed in male Kdm4b -FEs, while Pgk1 and Plac1 levels were reduced to <13% of those observed in controls ( Supplementary Fig. 11a ). In female Kdm4b -FEs, FISH analysis revealed that there were cells with Xist biallelic expression ( Supplementary Fig. 11b ). Although the expression level was slightly elevated (1.3-fold), X-linked genes were also significantly repressed in female Kdm4b -FEs ( Supplementary Fig. 11c ). These results showed that ectopic Xm- Xist derepression caused X-linked gene silencing and elimination of iXCI. To test the effects of iXCI disruption on postimplantation development, we conducted in vivo transplantation experiments. Interestingly, our results demonstrated that XCI on Xm during preimplantation did not affect developmental competence to term ( Kdm4b -FEs: 63.2% versus Egfp -FEs: 53.1%; Supplementary Fig. 11d,e ), suggesting that aberrant XCI in preimplantation embryos was restored during postimplantation development, probably through an automatic counting function. These results were consistent with the observation that the developmental competency of embryonic cloned embryos was high, despite the ectopic expression of Xist and the occurrence of global XCI ( Supplementary Fig. 12 ) [28] , [31] . Loss of XCI impairs the postimplantation development of PEs It is still unknown whether the embryonic lethality observed immediately after implantation in the majority of PEs (around 70–80%) can be attributed to the loss of dysregulation of X-linked genes or to loss of expression of autosomal paternally imprinted genes. Figure 2 showed that the percentage of Xist -positive cells in Kdm4b -PEs was significantly higher than that in Egfp -PEs. Thus, we reasoned that Kdm4b -PEs would be suitable for studying this long-standing question. We first performed a detailed analysis of Xm-XCI states in Kdm4b -PEs using IF against H3K27me3 and CDX2, a marker of the trophectoderm, in combination with Xist FISH, at the blastocyst stage. This analysis revealed that Xist -positive cells were significantly increased in the trophectoderm of Kdm4b -PEs, although the ratio of H3K27me3-positive cells was comparable to that of Egfp -PEs ( Fig. 5a–c and Supplementary Table 7 ). However, no significant difference was observed in the inner cell mass between groups ( Fig. 5a–c and Supplementary Table 7 ), indicating that loss of H3K9me3 in the maternal genome led to establishment of Xm-XCI as an imprinted Xp-XCI. Figure 5: Loss of Xm-XCI is the primary cause of developmental failure immediately after implantation in most PEs. ( a ) IF combined with FISH analysis of blastocysts in Egfp -PEs (upper panel) and Kdm4b -PEs (lower panel). CDX2-positive cells were identified as belonging to the trophectoderm (TE). Representative pictures of Z-sections. 4′,6-diamidino-2-phenylindole (DAPI) (blue), CDX2 (green), Xist (red) and H3K27me3 (white). Scale bars, 20 μm. The rates of cells with Xist (left) or H3K27me3 (right) in the inner cell mass (ICM) ( b ) and TE ( c ), respectively. n , number of embryos analysed. The number of cells analysed is shown in Supplementary Table 7 . * P <4.3 × 10 −23 (Fisher’s exact test). ( d ) Expression states and clustering analysis of imprinted genes. Sfmbt2 important for placentation and differentially expressed genes (asterisk) are shown. The scale bar indicates normalized values of log 2 . ( e ) Embryos with extra-embryonic tissues at E6.5 and E9.5 for Kdm4b - and Egfp -PEs, respectively. Upper and lower images indicate Egfp - and Kdm4b -PEs, respectively. Left and right column sides show E6.5 and E9.5, respectively. Scale bars, 200 μm (E6.5) and 500 μm (E9.5). ( f ) Summary of the developmental abilities of Kdm4b -PEs and Egfp -PEs at postimplantation stages (E6.5 and E9.5). Five and 12 independent recipients were analysed at E6.5 and E9.5, respectively. ( g , h ) Xist analysis in Rnf12- knockdown and control Kdm4b -PEs. Representative images of FISH analysis. Scale bars, 50 μm ( g ) and Xist expression states ( h ). ( i ) Expression of imprinted and X-linked genes in Rnf12 -knockdown and control Kdm4b -PEs. P -values were determined using Student’s t -tests. ( j ) Embryos with extra-embryonic tissues at E6.5 in Rnf12 -knockdown and control Kdm4b -PEs. Scale bars, 200 μm. ( k ) Summary of the developmental ability of Rnf12 -knockdown and control Kdm4b -PEs at E6.5. Five independent recipients were analysed. The P -values were determined using Fisher’s exact test. Full size image Next, we carried out transcriptome analysis in Egfp -PEs, Kdm4b -PEs and FEs using microarray. Clustering analysis based on gene expression patterns showed that all three groups could be distinguished clearly from each other ( Supplementary Fig. 13a ). Comparison of transcripts between Egfp -PEs and Kdm4b -PEs identified transcripts that were significantly differentially expressed: 671 transcripts were upregulated and 711 transcripts were downregulated ( P <0.05, Student’s t -test and>1.5-fold changes in Kdm4b -PEs). Chromosome distribution analysis showed that upregulated transcripts in Kdm4b -PEs were distributed across various chromosomes (2.33–7.23%; Supplementary Fig. 13b ). However, downregulated transcripts in Kdm4b -PEs were mostly concentrated on the X chromosome, which particularly involved the Xlr and Magea families (10.26%; Supplementary Fig. 13c–e ). Comparison of the imprinted genes between Egfp - and Kdm4b -PEs revealed that only six genes were significantly differentially expressed (paternally expressed genes: Impact and Fthl17 ; maternally expressed genes: Gnas , H13 , Xlr3b and Xlr4b ; Fig. 5d ). Clustering analysis based on the expression of imprinted genes showed that the expression levels in Kdm4b -PEs were similar to those in Egfp -PEs rather than to those of biparental embryos ( Fig. 5d ). Thus, H3K9me3 demethylation does not result in restoration of expression states in paternally expressed genes. We conducted in vivo transplantation experiments using Kdm4b -PEs. Surprisingly, at E6.5, the developmental rates of Kdm4b -PEs were markedly increased compared with those of Egfp -PEs ( Kdm4b -PEs: 90% versus Egfp -PEs: 35%; P <0.001, Fisher’s exact test; Fig. 5e,f ). At E9.5, although the stages of the recovered embryos varied, Kdm4b -PEs retained a significantly higher developmental ability compared with controls ( Kdm4b -PEs: 64.3% versus Egfp -PEs: 31.9%; P <0.002, Fisher’s exact test; Fig. 5e,f ). However, we did not rule out the possibility that the significant improvement in Kdm4b -PE development resulted from restoration of the expression levels of some imprinted genes. To determine whether the improvement in developmental competency could be attributed to the gain of XCI, we constructed Kdm4b +si- Rnf12 -PEs. In Kdm4b -PEs with si- Rnf12 at the blastocyst stage, Xist expression analysis by FISH revealed that Xist cloud signals in control Kdm4b -PEs were present in 51.9% of cells, while those in Rnf12 -knockdown Kdm4b -PEs were present in only 10% of cells, and most of the signals were pinpoint rather than cloud ( Fig. 5g,h and Supplementary Table 8 ). qPCR analysis showed that although Xist signals were significantly reduced in Kdm4b -PEs with si- Rnf12 (12.5% of the control on average), the expression levels of Impact , H13 and Gnas , which are expressed in response to ectopic Kdm4b expression ( Fig. 5d ), did not change when compared with those of controls ( Fig. 5i ). We further demonstrated that RNF12 depletion did not affect Tsix and Sfmbt2 expression levels in Kdm4b -PEs ( Fig. 5i ). These results clearly indicated that RNF12 depletion led to Xist downregulation in Kdm4b -PEs, without altering the features of PEs. Finally, in vivo transplantation experiments demonstrated that Xist repression by RNF12 depletion significantly inhibited developmental competency at E6.5 in Kdm4b -PEs ( Kdm4b +si-control: 84.2% versus Kdm4b +si- Rnf12 : 23.5%; P <0.0006, Fisher’s exact test; Fig. 5j,k ). Taken together, these results demonstrated that the developmental defects seen in PEs immediately after implantation could be attributed to the lack of XCI, but not to loss of expression of paternally expressed genes. In this study, we demonstrated that maternal imprinting of Xm, which protected against Xist activation by RNF12 in the preimplantation stages, was mediated by H3K9me3. Xm- Xist imprints are established during oogenesis and autosomal imprinting also occur in the phases [6] , [10] . In many imprinted genes, DNA methylation at the promoter regions is the primary regulator and H3K9me3 modifications overlap with these regions [32] . However, it is not clear why Xm- Xist regions are targeted by H3K9me3, but not by DNA methylation. One of the possibilities is that during primordial germ cell development, Xist must be silenced to activate the inactivated allele before inducing the expression of Dnmt3a / 3l , which encodes a de novo DNA methyltransferase that is activated during oogenesis [33] . Consistent with this concept, Xist repression begins in primordial germ cells at E10.5 (ref. 34 ). Thus, comparison of H3K9me3 states at promoter regions in non-growing oocytes with those in growing oocytes will greatly facilitate understanding of the molecular mechanisms of iXCI. We found that Kdm4b -, Egfp +TSA- and Kdm4b +TSA-PEs did not show complete XCI at the blastocyst stage as compared with female FEs. These results suggested that other repressive marks were imposed on Xm to silence Xm- Xist expression. Alternatively, removal of H3K9me3 may be incomplete because demethylation at RA regions was mild ( Fig. 4g ). However, it is not clear why RA regions show resistance against demethylation by KDM4B. As suggested in a previous study, this mechanism may be related to the three-dimensional structure of the A-repeat, which has been reported to constitute stable regions in the Xist transcript [35] . Further studies using ChIP-seq and/or chromatin-conformation capture sequencing technologies in preimplantation embryos are required for comprehensive understanding of Xist regulation. In ES cells, RNF12 induces Xist expression through degradation of REX1, which is required for suppression of Tsix [36] . Interestingly, we did not detect Tsix expression from the morula to the blastocyst stages in in vitro -fertilized (IVF) embryos, implying that the molecular mechanism of RNF12-mediated Xist activation differs between imprinted and randomly induced XCI. It is not known whether the role of RNF12 in Xist activation during the preimplantation stages was direct or indirect. Recent RNF12 studies reported the specific binding of RNF12 to Smad7 in mouse ES cells [37] , suggesting that signalling via transforming growth factor-β family members may be associated with imprinted Xist activation. In this study, we revealed the molecular mechanisms underlying imprinting of XCI and demonstrated the role of XCI in various types of embryo development in mice. Recent studies using somatic- and ES-cloned embryos revealed that aberrant Xist reprogramming is a major cause of developmental failure in cloned embryos [27] , [28] . We found that RNF12 was highly expressed in oocytes compared with somatic and ES cells (>80-fold). Moreover, we showed that H3K9me3 levels at Xist promoter regions were low in ES cells and that Xist expression in ES-cloned embryos depended on RNF12. These data provided the first evidence that RNF12 inhibited developmental reprogramming. Therefore, the use of RNF12-depleted oocytes as recipient cells would improve cloning efficiency. However, Xist activation in cloned embryos may be induced by factors other than RNF12, as supported by the observation that Xist was still expressed at ~40% of control levels, even after marked depletion of RNF12. Consistent with this notion, a recent study has demonstrated that RNF12 is dispensable for random XCI in vivo [38] . Xm- Xist derepression from the four-cell stage could rescue developmental defects in PEs. This finding demonstrated that the primary cause of developmental failure immediately after implantation was a lack of XCI, but not a lack of expression of paternally imprinted genes. We also tested whether Kdm4b -PEs could extend development; however, we did not observe extended Kdm4b -PE development after E9.5, implying that expression of paternally imprinted genes is required for subsequent development in PEs [11] , [12] . Our data resolved several long-standing unanswered questions about XCI during preimplantation in various types of embryos ( Supplementary Fig. 14 ). Moreover, given that injection of Kdm4b mRNA into PEs improved their developmental ability, genetic mutation leading to embryonic lethality could be rescued by transient expression of epigenomic modifiers during preimplantation phases. Embryo manipulations All mice were maintained and used in accordance with the Guidelines for the Care and Use of Laboratory Animals of the Japanese Association for Laboratory Animal Science and the National Research Institute for Child Health and Development (NRICHD) of Japan. All animal experiments were performed according to protocols approved by the Institutional Animal Care and Use Committee of the NRICHD (Permit Number: A2006-009). Adult female B6D2F1 mice were purchased from Clea Japan (Tokyo, Japan) and oocytes were collected following standard methods [27] . PEs were generated using Ca-free M16 medium containing 8 mM SrCl 2 and Cytochalasin B (5 μg ml −1 ) (Sigma-Aldrich, St Louis, MO, USA), and cultured KSOM (EMD Millipore, Darmstadt, Germany). Injection experiments (mRNA, short interfering RNA (siRNA) and nuclear transfer) were conducted using a Prime Tech Piezo drive (Sutter Instrument Company, Novato, CA, USA). To produce cloned embryos, nuclear-transferred oocytes were parthenogentically activated. Manipulated embryos were cultured to the developmental stages, as follows: 4-cell, 48 h; morula, 72 h; and blastocyst, 96 and 120 h after parthenogenetic activation or ICSI, respectively. All embryos were cultured at 37 °C in KSOM in an atmosphere containing 5% CO 2 . In the TSA experiment, the embryos were cultured for 24 h in activation and culture media containing 50 nM TSA (Sigma-Aldrich). IVF fertilization and nuclear transfer were performed following published procedures [27] . To determine the effects of ectopic KDM4B expression on Xist expression in cloned embryos, doxycycline was added to ES cell culture and KSOM medium to a final concentration of 2 μg ml −1 . Pseudopregnant ICR mice (Clea Japan) were used as embryo recipients. At E6.5, E9.5 and E18.5, the embryos were recovered from the uterus. In vitro mRNA synthesis The coding region of Kdm3a was amplified from mouse testis complementary DNA using PCR with KOD-Plus-Neo DNA polymerase (Toyobo, Osaka, Japan). Forward and reverse primers contained T7 promoter and poly(T) 120 sequences, respectively. A step-down PCR amplification method was used, following the manufacturer’s instructions (Toyobo). Poly(A)-containing PCR products were subjected to in vitro transcription using a mMESSAGE mMACHINE T7 ULTRA Kit (Life Technologies, Carlsbad, CA, USA), following the manufacturer’s instructions. To generate a Kdm4b DNA template for in vitro transcription, pCMV-SPORT6 containing the full-length Kdm4b mRNA was used as the PCR template (DNAFORM, Kanagawa, Japan, Clone ID 3490671). Egfp cDNA was cloned using the pGEM-T Easy Vector System (Promega, Madison, WI, USA) and transcribed in vitro using the mMESSAGE mMACHINE T7 ULTRA Kit (Life Technologies) following the manufacturer’s instructions. The concentrations of the mRNAs were adjusted to 150 ng ml −1 ( Egfp ), 550 ng ml −1 ( Kdm3a ), or 450 ng ml −1 ( Kdm4b ) to maintain a constant number of injected mRNA molecules. The primer sequences used for generating the templates for in vitro transcription are shown in Supplementary Table 9 . Rnf12 knockdown siRNA targeting Rnf12 (si-Rnf12 sense 5′-GAAGUCAAAUGGAUCGCUUTT-3′ A and antisense 5′-AAAGCGAUCCAUUUGACUUCTG-3′ GC, and the negative control siRNA (si-control: 4390846) were purchased from Life Technologies. The final concentration of each siRNA was 50 ng ml −1 . The siRNA was injected into MII oocytes using the Piezo drive and then incubated for 6–7 h in KSOM medium at 37 °C in an atmosphere containing 5% CO 2 before mRNA injection. For the NT experiment using Rnf12 -knockdown oocytes, oocytes were incubated for 5–6 h after siRNA injection, and NT was then conducted and activated as described above. Immunofluorescence Oocytes injected with mRNAs were subjected to ICSI. After 10–11 h, the zygotes were fixed with 2% paraformaldehyde (PFA) in PBS containing 0.1% polyvinyl alcohol (PBS-PVA) for 15 min at room temperature (RT). Zygotes were then permeabilized using 0.2% Triton X-100 in PBS-PVA for 15 min at RT and blocked in 1% BSA in PBS-PVA for 1 h at RT. The primary antibodies used in the assay were as follows: anti-H3K9me3 (ab8898, 1:500 dilution, Abcam, Cambridge, UK), anti-H3K9me2 (ab1220, 1:500, Abcam) and anti-H3K27me3 (07-449, 1:150, EMD Millipore). The primary antibodies were diluted with blocking solution (PBS-PVA containing 1% BSA) and the embryos were incubated overnight at 4 °C. After washing in blocking solution, the embryos were incubated for 1 h at RT with Alexa Flour 634- or 546-conjugated anti-mouse or anti-rabbit IgG secondary antibodies (1:500, Life Technologies). After the embryos were washed, the nuclei were stained with 1 μg ml −1 4′,6-diamidino-2-phenylindole and the embryos were placed on a glass slide and observed with a LSM510 laser scanning confocal microscope (Carl Zeiss, Oberkochen, Germany). Signal intensities of maternal and paternal pronuclei were calculated using NIH ImageJ software ( http://rsb.info.nih.gov/ij/ ). In Rnf12- knockdown experiments, one-cell and four-cell PEs were fixed at 10–11 h (18–19 h after siRNA injection) and 48 h after activation, respectively. Anti-RNF12 (1:500, Abnova, Taipei, Taiwan) and Alexa Fluor 488-conjugated anti-mouse IgG antibodies (1:500, Life Technologies) were used as the primary and secondary antibodies, respectively. Rnf12- knockdown and negative-control PEs were observed under the same conditions, to assess knockdown efficiency. Signal intensities were calculated using ImageJ software. Fluorescent in situ hybridization The zona pellucida of embryos was removed using acid Tyrode solution (Sigma-Aldrich) and then fixed and permeabilized with 2% PFA-PVA containing 0.25% Triton X-100 for 10 min on ice. The samples were placed on glass slides, evaporated to dryness, dehydrated sequentially in 70 and 100% ethanol and then air-dried. Hybridization buffer containing an Xis t probe (provided by T. Sado) was prepared using a Nick Translation Kit (Abbott, Abbott Park, IL, USA) and Cy3-dUTP (GE Healthcare Life Sciences, Fairfield, CT, USA) and was then applied to the slides. The slides were then incubated and washed as previously described [26] . Fluorescence was visualized using the LSM510. IF combined with FISH The zona pellucida of embryos was removed using acid Tyrode solution (Sigma-Aldrich) and fixed with 2% PFA-PVA for 15 min at RT in four-well dishes. The fixed samples were permeabilized with 0.5% Triton X-100 in PBS-PVA for 20 min on ice. After washing with PBS-PVA, the samples were blocked in 1% BSA-PBS-PVA containing 1.3 U ml −1 RNaseOUT (Life Technologies) for 30 min at RT. After washing, the embryos were incubated with primary antibodies (anti-CDX2 (BioGenex, San Ramon, CA, USA), diluted 1:30 and anti-H3K27me3 diluted 1:150 in blocking buffer containing 1.3 U ml −1 RNaseOUT) for 1 h at RT. Secondary antibody reactions were performed as described above. The samples were placed on glass slides, evaporated to dryness, dehydrated sequentially in 70 and 100% ethanol and air dried. The samples were then analysed by FISH according to the procedures described above. Analysis of IF combined with FISH data Xist cloud signals detected in three-dimensional images using Z -sections of the LSM Image Browser (Carl Zeiss) were judged as positive. Only cells that did not overlap at interphase were used in the analysis. Biallelic expression was defined as cells with two Xist cloud spots. Statistical analysis was performed using Fisher’s exact test. Gene expression analysis Total RNA was extracted using an RNeasy Micro Kit (Qiagen, Venlo, The Netherlands) and treated with DNase following the manufacturer’s instructions. mRNAs were reverse transcribed using an oligo(dT) primer and SuperScriptIII Reverse Transcriptase (Life Technologies). For quantitative gene expression analysis with high specificity, TaqMan probes (Life Technologies) were used in all assays. In four-cell stage embryos, Xist was assayed in triplicate and only the samples that were detected in two or three replicates were judged as positive. In morulae and blastocysts, expression of target genes was assayed in duplicate. Gapdh was used as the internal control in the four-cell-stage assays and Rnf12 was used in the time-lapse assays. Gapdh and Actb (encoding β-actin) were used as internal controls at the morula and blastocyst stages. For normalization of qPCR analysis ( Fig. 2b,g ), the expression levels of all embryos were normalized to the average expression levels of Egfp -PEs. The TaqMan probes and primer sets used in this study are shown in Supplementary Table 8 . Generation of Kdm4b -inducible ES cell lines and ES cell culture The XhoI- and ClaI-linearized pGEM-IRES-EGFP plasmids were inserted into the cognate sites of pPB-CAG-EBNX (provided by A. Bradley) to generate pPB-CAG-IRES-EGFP. A Tet3G fragment with BglII and XhoI cleavage sites was amplified from a pEF1a-Tet3G template (Clontech Laboratories, Mountain View, CA, USA) using PCR and inserted into pPB-CAG-IRES-EGFP, generating the vector pPB-CAG-Tet3G-IRES-EGFP. The XhoI and BamHI cleavage sites in pPB-UbC (provided by A. Bradley) were replaced with the p-TRE3G multiple cloning sites (Clontech). The Kdm4b coding sequence, with terminal ClaI and BamHI cleavage sites, was amplified by PCR and inserted into the corresponding sites of pPB-TRE3G, yielding pPB-TRE-Kdm4b. The NCH.4.6 male mouse ES cell line (C57B6/N × C57B6/N), which had a normal karyotype, was electroporated with pPB-TRE-Kdm4b, pPB-CAG-Tet3G-IRES-EGFP and pCMV-hyPBase (provided by A. Bradley). All ES cells used in this study were cultured in knockout DMEM (Life Technologies) containing recombinant human leukemia inhibitory factor culture supernatant for mouse ES cell culture (Wako Pure Chemical Industries, Ltd, Osaka, Japan), as well as GlutaMAX, 2-mercaptoethanol, non-essential amino acids and 15% KSR (all from Life Technologies). Doxycycline (2 μg ml −1 ; Sigma-Aldrich) was added to ES cell culture medium to induce ectopic KDM4B expression. Western blotting Cells were extracted using a stock lysis buffer containing 1 M Tris–HCl, 5 M NaCl, 10% Triton-X and protease inhibitors, and were subjected to e-PAGEL (ATTO, Amherst, NY, USA) electrophoresis. The membranes were washed in TBS containing 0.1% Tween 20 (TBS-T) and blocked in 5% skim milk in TBS-T for 1 h. The membranes were incubated with anti-KDM4B antibodies (1:500 dilution; Active Motif, Carlsbad, CA, USA) overnight at 4 °C, washed and incubated with a rabbit horseradish peroxidase-conjugated secondary antibody (1:5,000 dilution; Sigma-Aldrich) for 1 h at RT. Immunoblottings were visualized using SuperSignal chemiluminescent substrate (Thermo Scientific, Waltham, MA, USA) and an ImageQuant LAS4000 system (GE Healthcare). After capturing the images, the membranes were washed with WB Stripping Buffer (Nacalai Tesque, Kyoto, Japan) for 10 min, washed with TBS-T and incubated with an anti-β-actin antibody conjugated to fluorescein isothiocyanate (1:2,000 dilution; Sigma-Aldrich) for 1 h at RT. ChIP analysis of K4B-ES cells Trypsinized feeder-free ES cells (2 × 10 7 ) were collected and fixed with 1% formaldehyde. The cells were resuspended in SDS lysis buffer (ChIP Reagent, Nippon Gene Co., Ltd.) and the lysate was sonicated to fragment chromatin using a S220 Focused-ultrasonicator (Covaris, Woburn, MA, USA). The chromatin was purified by centrifugation and immunoprecipitated with Protein A-beads (Veritas Life Sciences, Ribeirão Preto, Brazil) conjugated to anti-H3K9me3 antibodies (Abcam: ab8898) or rabbit IgG (Abcam: ab37415) in Buffer A with protease inhibitor (LowCell ChIP kit, Diagenode, Denville, NJ, USA) overnight at 4 °C. The chromatin beads were washed with Buffers A and C (LowCell ChIP kit). After washing, the chromatin beads were incubated in ChIP direct elution buffer (ChIP Reagent) for 6 h at 65 °C, following incubation with 2 μl proteinase K (20 mg0 ml −1 ) for 2 h at 55 °C. The DNA immunoprecipitated from the supernatant was purified using Agencourt AMPure XP beads (Beckman Coulter, Inc., Pasadena, CA, USA) according to the manufacturer’s instructions. ChIP combined with deep sequencing ChIP-Seq libraries were prepared using the NEBNext ChIP-Seq Library Prep Master Mix Set and Multiplex Oligos from Illumina (New England BioLabs Inc., Ipswich, MA, USA) according to the manufacturer’s instructions. Ten nanograms of ChIP or input DNA was subjected to end repair, dA-tailing and adaptor ligation, and amplified using nine cycles of PCR. The final library size was checked using a 2100 Bioanalyzer (Agilent Technologies, Santa Clara, CA, USA). After the concentration of each library was determined using qPCR with a KAPA Library Quantification Kit-Illumina/Universal system (KK4824, Kapa Biosystems, Wilmington, MA, USA), the libraries were sequenced using the HiSeq 1000 sequencing system (Illumina, San Diego, CA, USA) to generate 100 bp × 2 paired-end data. ChIP-seq data analysis Reads from each sample were first trimmed by removing adapter sequences and low-quality bases at ends using Trimmomatic 0.22 ( http://www.usadellab.org/cms/index.php?page=trimmomatic ). Approximately 115 million reads for each of the ChIP and input libraries were aligned to the mouse reference genome (mm10: http://genome.ucsc.edu/cgi-bin/hgGateway ) using the Burrows-Wheeler Aligner 0.6.2. Uniquely mapped reads were selected using a custom script, converted from SAM to BAM format using SAMtools 0.1.18 and processed using Picard 1.83 to mark PCR duplicates. Reads with a mapping quality of <20 were removed using SAMtools 0.1.18. The resulting BAM files (a pair of files for ChIP and input libraries) were visualized using the Integrative Genomics Viewer ( http://www.broadinstitute.org/igv/ ) and subjected to peak detection using the MACS algorithm implemented in Avadis NGS software (Agilent). In scatter plot analysis using 1 and 15 K4B-ES cell lines, the numbers of mapped reads were counted for 10,000-bp windows (with a sliding size of 5,000 bp). To adjust for differences in total amount of reads, the number of mapped reads in each window was transformed into reads per million format. Calculation methods are available on request. ChIP-qPCR analysis of sperm Sperm were obtained from BDF1 mice aged 9–12 weeks. Preparation of sperm chromatin was performed according to published protocols with modifications [39] , [40] . For each native ChIP experiment, 5 × 10 7 sperm were used. Sperm were washed twice with PBS. The pellet was suspended in PBS containing 0.5% Triton-X, 10 mM dithiothreitol (DTT) and protease inhibitor (Diagenode), and incubated on ice for 1.5 h. After washing with PBS, pelleted sperm nuclei were suspended in 400 μl PBS containing 1 mM CaCl 2 and 1 mM DTT, and incubated for 5 min at 37 °C. After incubation, 1 μl (2 × 10 6 gel units per ml) micrococcal nuclease (New England BioLabs) was added to the nuclei, which were then incubated for 5 min at 37 °C. EDTA was added to a concentration of 0.5 mM and solubilized chromatin was clarified by centrifugation for 15 min at 15,000 r.p.m. at 4 °C. The pellets were suspended in PBS containing CaCl 2 and DTT (at the same concentrations as used above), and treated again with micrococcal nuclease. To examine whether H3K9me3-modified nucleosomes were present in sperm chromatin, soluble (chromatin) and insoluble (pellet) fractions were subjected to western blotting using anti-H3K9me3 antibodies (ab8898; 1:1,000), as described above. Chromatin was incubated with Protein A beads conjugated to anti-H3K9me3 antibodies (ab8898) or rabbit IgG (ab37415) overnight at 4 °C in ChIP buffer (40 mM Tris–HCl, pH 7.5, 1 M NaCl and 10 mM EDTA). Pelleted beads were washed twice with Buffer 1 (50 mM Tris–HCl, pH 7.5, 500 mM NaCl and 10 mM EDTA) and Buffer 2 (50 mM Tris-HCL, pH 7.5, 300 mM NaCl and 10 mM EDTA). The pelleted beads were suspended in ChIP direct elution buffer and incubated with proteinase K for 2 h at 37 °C. The immunoprecipitated DNA was then purified using Agencourt AMpure XP beads. ChIP-qPCR analysis was performed according to published methods using SYBR Green [39] . The sequences of each primer set are listed in Supplementary Table 9 . eChIP-quantitative qPCR The zona pellucidae of the embryos were removed by acid Tyrode’s solution and washed in PBS containing 0.1% PVA. The embryos were suspended in PBS containing 0.5% Triton-X, 0.5 mM DTT and protease inhibitor, and incubated on ice for 30 min. After incubation, 1 mM CaCl 2 was added to the buffer and samples were incubated for 5 min at 37 °C. After incubation, 0.5 μl (2 × 10 6 gel units per ml) micrococcal nuclease (New England BioLabs) was added to the nuclei, which were then incubated for 5 min at 37 °C. EDTA was added to a concentration of 0.5 mM and solubilized chromatin was clarified by centrifugation at 15,000 r.p.m. for 15 min at 4 °C. The same procedures were repeated one more time. Chromatin was incubated with Protein A beads conjugated to anti-H3K9me3 antibodies (ab8898) or rabbit IgG (ab37415), prepared as described above, overnight at 4 °C in ChIP buffer (40 mM Tris–HCL, pH 7.5, 1 M NaCl and 10 mM EDTA). Pelleted beads were washed twice with Buffer 1 (50 mM Tris–HCL, pH 7.5, 500 mM NaCl and 10 mM EDTA) and then with Buffer 2 (50 mM Tris–HCL, pH 7.5, 300 mM NaCl and 10 mM EDTA). The pelleted beads were then suspended in ChIP direct elution buffer and incubated with proteinase K for 2 h at 55 °C. The immunoprecipitated DNA was then purified using Agencourt AMpure XP beads. Eluted DNA (20 μl) was divided into two aliquots; one (4 μl) was used for a SYBR Green assay targeting a major satellite and the other (16 μl) was subjected to pre-amplification using a Single Cell-to-CT kit (Ambion, Austin, TX, USA) according to the manufacturer’s instructions. The number of PCR cycles at the pre-amplification step was 20. The primer and probe sequences used are shown in Supplementary Table 9 . Microarray analysis Five Egfp -PE, Kdm4b -PE and IVF blastocysts (120 h) were lysed using ISOGEN (Nippongene) and RNA was extracted by phenol–chloroform and isopropanol precipitation. cDNA was synthesized using the Ovation RNA Amplification System V2 kit (NuGEN, West Cumbria, UK) and hybridized with SurePrint G3 Mouse GE 8x60K Microarray (Agilent Technologies). Analysis was conducted using GeneSpringV12.5 (Agilent Technologies). Transcripts were considered to be expressed if raw values were >100 and a flag was present in at least one of the groups. How to cite this article : Fukuda, A. et al. The role of maternal-specific H3K9me3 modification in establishing imprinted X-chromosome inactivation and embryogenesis in mice. Nat. Commun. 5:5464 doi: 10.1038/ncomms6464 (2014). Accession codes: The original data for the microarray have been deposited in the GEO at http://www.ncbi.nlm.nih.gov/geo/ (accession number: GSE53662 ). The original data of ChIP-seq have been deposited in DDBJ at http://cibex.nig.ac.jp/index.jsp with accession number: DRA001041 .